Hepatocyte Toll-like receptor 4 regulates obesity-induced inflammation and insulin resistance Chronic low-grade inflammation is a hallmark of obesity and thought to contribute to the development of obesity-related insulin resistance. Toll-like receptor 4 (Tlr4) is a key mediator of pro-inflammatory responses. Mice lacking Tlr4s are protected from diet-induced insulin resistance and inflammation; however, which Tlr4-expressing cells mediate this effect is unknown. Here we show that mice deficient in hepatocyte Tlr4 (Tlr4 LKO ) exhibit improved glucose tolerance, enhanced insulin sensitivity and ameliorated hepatic steatosis despite the development of obesity after a high-fat diet (HFD) challenge. Furthermore, Tlr4 LKO mice have reduced macrophage content in white adipose tissue, as well as decreased tissue and circulating inflammatory markers. In contrast, the loss of Tlr4 activity in myeloid cells has little effect on insulin sensitivity. Collectively, these data indicate that the activation of Tlr4 on hepatocytes contributes to obesity-associated inflammation and insulin resistance, and suggest that targeting hepatocyte Tlr4 might be a useful therapeutic strategy for the treatment of type 2 diabetes. The increasing incidence of obesity and associated diseases has become a worldwide health problem. One hallmark of obesity is chronic, low-grade inflammation, characterized by increased pro-inflammatory cytokines in the circulation and tissues [1] , [2] . In addition, this elevated inflammatory status plays an important role in the development of insulin resistance [3] . It has been shown that obese subjects and diet-induced animal models have increased circulating lipopolysaccharide (LPS) levels [4] , [5] . LPS is the outer membrane glycolipid of gram-negative bacterial and it can initiate a potent immune response through its interaction with the cell surface receptor, Toll-like receptor 4 (Tlr4). The activation of Tlr4 signalling pathway leads to the generation of pro-inflammatory cytokines through the upregulation of several transcription factors, including Nuclear Factor-κB (NF-κB), Activated Protein 1 (AP-1) and Interferon Regulatory Factors (IRFs) [6] . Thus, by blocking Tlr4-mediated inflammatory signalling, mice lacking Tlr4 show greatly attenuated diet-induced inflammation and insulin resistance [7] , [8] , [9] , [10] , [11] . However, Tlr4 is widely expressed throughout the body and the exact Tlr4-expressing cell types that contribute to the development of metabolic disorders are unknown. The liver is a key insulin-responsive tissue and is actively involved in maintaining whole-body glucose and lipid metabolism. Accumulating evidence suggests a role of hepatocyte-initiated inflammation in the development of insulin resistance. Specifically, hepatocyte activation of the inhibitor of NF-κB kinase beta subunit (IKKβ)/NF-κB in mice causes hepatic and systemic insulin resistance, as well as increased hepatic production of inflammatory cytokines [12] . In addition, mice lacking IKKβ in hepatocytes maintain insulin sensitivity and glucose tolerance in the liver despite the development of obesity [13] . Notably, the expression of Tlr4 in hepatocytes, including murine hepatoma cell lines [14] and primary hepatocytes from rodents [14] , [15] , [16] and humans [17] , [18] , [19] , [20] is well documented. However, the role of hepatocyte Tlr4 in obesity and related metabolic disorders remains to be determined. M1 macrophages (or classically activated macrophages) are one of the major cell types that produce various pro-inflammatory cytokines and chemokines. The role of macrophage-mediated inflammation in the pathogenesis of insulin resistance has been widely investigated [21] . The results of two recent studies using bone marrow transplantation techniques to investigate the role of hematopoietic Tlr4 in diet-induced metabolic disorders reported disparate effects [22] , [23] . As bone marrow-derived cells include not only macrophages but also other immune cells, including dendritic cells, B cells and T cells, the exact role of macrophage Tlr4 in diet-induced inflammation and insulin resistance is unclear. To directly address the tissue-specific role Tlr4 in diet-induced obesity and associated metabolic abnormalities, we generated two mouse models that are deficient in either hepatocyte (Tlr4 LKO ) or myeloid cell (Tlr4 ΔmΦ ) Tlr4. Our findings show that after high-fat diet (HFD) feeding, Tlr4 LKO mice become obese, but have markedly improved insulin sensitivity and significantly attenuated inflammatory response in both adipose tissue and in the circulation. However, Tlr4 ablation in myeloid cells does not ameliorate HFD-induced insulin resistance. Taken together, these data indicate an important role of hepatocyte Tlr4 in the regulation of obesity-associated metabolic disorders. Generation and validation of the Tlr4 fl/wt mice To investigate the tissue-specific role of Tlr4, we generated a mouse model harbouring a loxP-modified Tlr4 allele (Tlr4 fl/wt ). The gene-targeting strategy was shown in Supplementary Fig. 1a . Tlr4 fl/wt mice were mated with each other, and the offspring were genotyped for either the wild-type (WT) or floxed allele by PCR using genomic DNA from mouse tails ( Supplementary Fig. 1b ). To validate the utility of this mouse model, we generated whole-body Tlr4 null mice by crossing Tlr4 fl/wt mice with Zona Pellucida 3-Cre (Zp3-cre) mice [24] . Heterozygous Tlr4 (Tlr4 +/− ) mice from this breeding were used to generate homozygous Tlr4 null (Tlr4 KO ) mice and WT littermates. It has been reported that Tlr4 mediates the production of inflammatory cytokines in LPS-induced endotoxin shock [6] , [25] , [26] . To assess the inflammatory response in WT and Tlr4 KO mice, we treated mice with intraperitoneal injections of LPS. Expectedly, Tlr4 deletion in mice led to >90% reduction in plasma levels of tumour necrosis factors α (Tnfα) compared with that of WT mice ( Supplementary Fig. 1c,d ). These findings indicate that the Cre-conditional Tlr4 null allele undergoes Cre-mediated recombination and deletion. Hepatocyte Tlr4 deficiency attenuates insulin resistance To examine the metabolic role of Tlr4 in the liver, we generated liver-specific Tlr4 null mice (Tlr4 LKO ) by crossing Tlr4 fl/fl mice to mice bearing an Albumin-Cre transgene. Primary hepatocytes isolated from Tlr4 LKO mice showed the presence of the Tlr4 Δ allele ( Fig. 1a ) and a significant reduction of Tlr4 mRNA expression ( Fig. 1b ). Next, we examined the contribution of hepatocyte Tlr4 in LPS-induced inflammatory response. After LPS administration, Tlr4 LKO mice exhibited significantly reduced plasma concentration of Tnfα, showing an ∼ 25% decrease compared with chow-fed Tlr4 fl/fl mice ( Fig. 1c,d ). This is consistent with a previous report that Tlr4 expression in hepatocyte mediates a low response to LPS [17] . 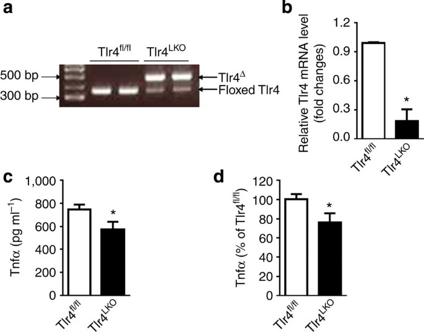Figure 1: Generation of mice deficient in hepatocyte Tlr4. (a) PCR analysis of genomic DNA isolated from primary hepatocytes of Tlr4fl/fland Tlr4LKOmice. (b) qPCR analysis of Tlr4 mRNA expression in primary hepatocytes isolated from chow-fed mice. (c) LPS (1 mg kg−1body weight) was injected intraperitoneally to chow-fed mice. Blood was collected 1.5 h after LPS administration and plasma Tnfα levels were measured by the MILLIPLEX Mouse Cytokine/Chemokine assay (n=5–8). (d) Levels are presented as a percentage relative to Tlr4fl/fllevels. *P<0.05, compared between Tlr4LKOand Tlr4fl/flmice (Student’st-test). All data are presented as means±s.e.m. Figure 1: Generation of mice deficient in hepatocyte Tlr4. ( a ) PCR analysis of genomic DNA isolated from primary hepatocytes of Tlr4 fl/fl and Tlr4 LKO mice. ( b ) qPCR analysis of Tlr4 mRNA expression in primary hepatocytes isolated from chow-fed mice. ( c ) LPS (1 mg kg −1 body weight) was injected intraperitoneally to chow-fed mice. Blood was collected 1.5 h after LPS administration and plasma Tnfα levels were measured by the MILLIPLEX Mouse Cytokine/Chemokine assay ( n =5–8). ( d ) Levels are presented as a percentage relative to Tlr4 fl/fl levels. * P <0.05, compared between Tlr4 LKO and Tlr4 fl/fl mice (Student’s t -test). All data are presented as means±s.e.m. Full size image To investigate the role of hepatocyte Tlr4 in diet-induced obesity and associated metabolic disorders, we fed Tlr4 fl/fl and Tlr4 LKO mice either chow or HFD for 12 weeks. Compared with chow-fed mice, HFD-fed mice became obese ( Supplementary Fig. 2a ). Regardless of diets, we observed similar body weight curves ( Supplementary Fig. 2a ) and comparable epididymal fat pad mass ( Supplementary Fig. 2b ) in both genotypes. Consistently, haematoxylin and eosin (H&E) staining showed no differences in adipocyte size or morphology between Tlr4 fl/fl and Tlr4 LKO mice on HFD ( Supplementary Fig. 2c ). In addition, HFD-fed Tlr4 fl/fl and Tlr4 LKO mice had similar plasma leptin concentrations ( Supplementary Fig. 2d ). Collectively, these data indicate that the loss of Tlr4 from hepatocytes does not affect the development of HFD-induced obesity. Since obesity is frequently associated with insulin resistance, we next examined whether hepatocyte-specific Tlr4 deletion in mice alters systemic insulin sensitivity. Compared with chow-fed animals, mice of both genotypes on HFD became hyperglycemic and hyperinsulinemic ( Supplementary Fig. 3a,b ). Despite similar blood glucose levels under fasted conditions and comparable plasma insulin levels under either fed or fasted states, obese Tlr4 LKO mice had slightly but significantly lower blood glucose levels under fed conditions ( Supplementary Fig. 3a ). We next performed glucose tolerance (GTT) and insulin tolerance tests (ITT). Expectedly, HFD-fed mice were glucose-intolerant and insulin-resistant compared with chow-fed animals ( Fig. 2a,b and Supplementary Fig. 3c,d ). Interestingly, HFD-fed Tlr4 LKO mice showed significantly reduced blood glucose levels after the injection of a bolus of glucose ( Fig. 2a ), indicating improved glucose tolerance. Additionally, the plasma insulin levels during the GTT were significantly lower in Tlr4 LKO mice ( Fig. 2c ). Moreover, HFD-fed Tlr4 LKO mice exhibited significantly decreased blood glucose concentrations at 60 and 120 min after insulin injection ( Fig. 2b ), suggesting enhanced insulin sensitivity. 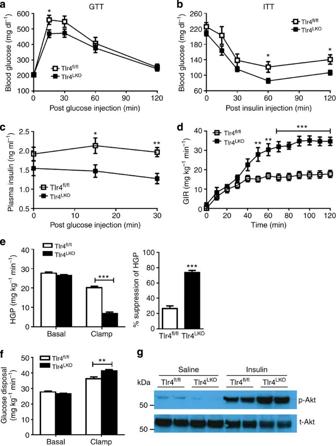Figure 2: Hepatocyte Tlr4 promotes HFD-induced insulin resistance in mice. (a) Glucose tolerance test (GTT, 1.2 mg g−1BW,n=9–11) in 5-h fasted HFD-fed mice. (b) Insulin tolerance test (ITT, 1.5 mU g−1BW,n=8–10) in 5-h fasted HFD-fed mice. (c) Glucose-stimulated insulin secretion in overnight fasted mice after 8 weeks of HFD feeding. Glucose (2 mg g−1BW) were injected intraperitoneally and plasma insulin concentrations were measured at the indicated time points (n=6–7). (d–f) After 16 weeks HFD feeding, hyperinsulinemic-euglycemic (10 mU kg−1min−1, 150 mg dl−1, respectively) clamps of 120 min were performed in conscious, chronically catheterized, 4–5-h fasted Tlr4fl/fland Tlr4LKOmice (n=6–7). (d) Glucose infiltration rate (GIR) during the 120-min clamp experiment. (e,f) Basal and insulin-stimulated (clamp steady-state (t=80–120 min)) hepatic glucose production (e, HGP) and glucose disposal rate (f). (g) Western blotting of insulin-stimulated Akt phosphorylation in epididymal fat pad from HFD-fed Tlr4fl/fland Tlr4LKOmice. Representative western blot images are shown. *P<0.05, **P<0.01, ***P<0.001, compared between Tlr4fl/fland Tlr4LKOmice (Student’st-test). All data are presented as means±s.e.m. Figure 2: Hepatocyte Tlr4 promotes HFD-induced insulin resistance in mice. ( a ) Glucose tolerance test (GTT, 1.2 mg g −1 BW, n =9–11) in 5-h fasted HFD-fed mice. ( b ) Insulin tolerance test (ITT, 1.5 mU g −1 BW, n =8–10) in 5-h fasted HFD-fed mice. ( c ) Glucose-stimulated insulin secretion in overnight fasted mice after 8 weeks of HFD feeding. Glucose (2 mg g −1 BW) were injected intraperitoneally and plasma insulin concentrations were measured at the indicated time points ( n =6–7). ( d – f ) After 16 weeks HFD feeding, hyperinsulinemic-euglycemic (10 mU kg −1 min −1 , 150 mg dl −1 , respectively) clamps of 120 min were performed in conscious, chronically catheterized, 4–5-h fasted Tlr4 fl/fl and Tlr4 LKO mice ( n =6–7). ( d ) Glucose infiltration rate (GIR) during the 120-min clamp experiment. ( e , f ) Basal and insulin-stimulated (clamp steady-state ( t =80–120 min)) hepatic glucose production ( e , HGP) and glucose disposal rate ( f ). ( g ) Western blotting of insulin-stimulated Akt phosphorylation in epididymal fat pad from HFD-fed Tlr4 fl/fl and Tlr4 LKO mice. Representative western blot images are shown. * P <0.05, ** P <0.01, *** P <0.001, compared between Tlr4 fl/fl and Tlr4 LKO mice (Student’s t -test). All data are presented as means±s.e.m. Full size image We then performed hyperinsulinemic-euglycemic clamps in body weight-matched animals ( Supplementary Fig. 4a ) to assess the specific tissues that are responsible for improved glucose homeostasis in HFD-fed Tlr4 LKO mice. We found that the glucose infusion rate needed to maintain euglycemia (~ 150 mg dl −1 in Supplementary Fig. 4b ) was markedly increased in Tlr4 LKO mice compared with their littermate controls ( Fig. 2d ), indicating improved whole-body insulin sensitivity. Strikingly, hepatic glucose production under hyperinsulinemic clamp conditions was dramatically suppressed in Tlr4 LKO mice ( Fig. 2e ). In addition, insulin-stimulated glucose disposal was slightly, but significantly, increased in Tlr4 LKO mice compared with Tlr4 fl/fl mice ( Fig. 2f ). Insulin sensitivity in adipose tissue was assessed by insulin-stimulated phosphorylated Protein Kinase B (also known as Akt) expression. After an injection of insulin, pAkt levels were greatly increased in the adipose tissue of Tlr4 LKO mice ( Fig. 2g ), indicating enhanced insulin sensitivity. These data suggest that hepatocyte-specific Tlr4 deficiency attenuates diet-induced whole-body insulin resistance, mainly in the liver and adipose tissue. Consistent with our findings, Uchimura et al. [27] recently reported that hepatic Tlr4 plays an important role in regulating glucose metabolism and insulin sensitivity in mice. Hepatocyte Tlr4 deficiency attenuates inflammation Given the close association between obesity, insulin resistance and inflammation, we examined the expression of several inflammatory markers in the liver and white adipose tissue (WAT) of HFD-fed mice. We found that both liver and epididymal WAT of Tlr4 LKO mice had reduced interleukin-1beta (IL-1β) and IL-6 mRNA expression ( Fig. 3a,c ). However, significant decreases in mRNA expression of Tnfα, monocyte chemotactic protein 1 (Mcp1) and suppressor of cytokine signalling 3 (Socs3) were only seen in the WAT of Tlr4 LKO mice ( Fig. 3a ). Moreover, mRNA expression of Cd11c, a M1 macrophage marker, tended to be reduced in the WAT of HFD-fed Tlr4 LKO mice ( Fig. 3a ). However, markers for anti-inflammatory M2 macrophages (arginase 1 (Arg1), mannose receptor, C type 1 (Mrc1) and C-type lectin domain family 10, member A (Clec10a)) were comparable between two genotypes ( Fig. 3a ). 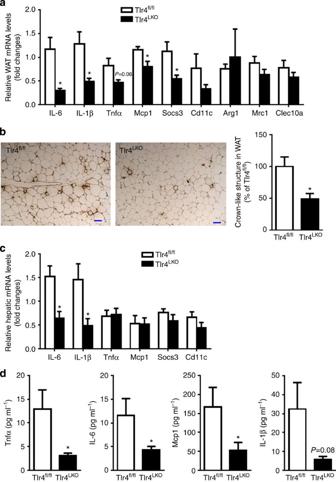Figure 3: Hepatocyte Tlr4 stimulates obesity-related tissue and systemic inflammation in mice. (a) qPCR analysis of genes in epididymal WAT of HFD-fed mice (n=4–6). (b) Mac2 staining of epididymal WAT sections prepared from mice on HFD and quantification of crown-like structures. Scale bars, 100 μm. (c) qPCR analysis of genes in the liver of HFD-fed mice (n=4–6). (d) Plasma Tnfa, IL-6, IL-1β and Mcp1 levels in mice fed HFD (n=12–16 for Tnfα and Mcp1;n=9–10 for IL-1β and IL-6). *P<0.05, compared between Tlr4fl/fland Tlr4LKOmice (Student’st-test). All data are presented as means±s.e.m. Figure 3: Hepatocyte Tlr4 stimulates obesity-related tissue and systemic inflammation in mice. ( a ) qPCR analysis of genes in epididymal WAT of HFD-fed mice ( n =4–6). ( b ) Mac2 staining of epididymal WAT sections prepared from mice on HFD and quantification of crown-like structures. Scale bars, 100 μm. ( c ) qPCR analysis of genes in the liver of HFD-fed mice ( n =4–6). ( d ) Plasma Tnfa, IL-6, IL-1β and Mcp1 levels in mice fed HFD ( n =12–16 for Tnfα and Mcp1; n =9–10 for IL-1β and IL-6). * P <0.05, compared between Tlr4 fl/fl and Tlr4 LKO mice (Student’s t -test). All data are presented as means±s.e.m. Full size image Next, we examined macrophage content in the fat pads of HFD-fed mice by Mac2 immunohistochemistry staining. We found that the level of infiltrated macrophages was greatly reduced in the fat pads of Tlr4 LKO mice ( Fig. 3b ). Furthermore, circulating concentrations of pro-inflammatory cytokines, including Tnfα, IL-6, IL-1β and Mcp1, were greatly reduced in obese Tlr4 LKO mice compared with that of HFD-fed controls ( Fig. 3d ). Hepatocyte Tlr4 deficiency attenuates hepatic steatosis Fat accumulation in the liver is a manifestation of obesity-related metabolic syndrome. Indeed, while HFD caused a significant increase in liver weights in mice of both genotypes ( Fig. 4a ), the weight gain was significantly less in livers from HFD-fed Tlr4 LKO mice. Furthermore, livers from HFD-fed Tlr4 LKO mice showed decreased triglyceride and cholesterol contents ( Fig. 4b,c ). Moreover, qPCR analyses of liver tissues indicated that mRNA expression of genes involved in de novo lipogenesis was attenuated (acetyl CoA carboxylase 1 (Acc1), fatty acid synthase (Fas) and stearoyl CoA desaturase 1 (Scd1)) ( Fig. 4d ). However, genes involved in gluconeogenesis (forkhead box protein O1 (Foxo1) and phosphoenolpyruvate carboxykinase (Pepck)) and fatty acid oxidation (acyl-CoA oxidase 1 (Acox1)) were unchanged ( Fig. 4d ). In addition, plasma levels of alanine transaminase (ALT) and aspartate aminotransferase (AST), two markers of liver damage, were decreased ( Fig. 4e ). These findings suggest that liver injury associated with the development of non-alcoholic fatty liver disease was attenuated in obese Tlr4 LKO mice. However, comparable plasma concentrations of triglyceride, cholesterol and non-esterified fatty acid (NEFA) were observed in mice on HFD ( Supplementary Fig. 5a–c ). 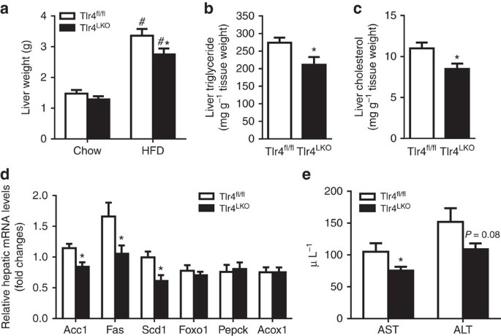Figure 4: Hepatocyte Tlr4 promotes the development of hepatic steatosis and liver injury in mice. (a) Liver weight in mice fed either chow (n=8) or HFD (n=10) for 12 weeks. (b) Liver triglyceride contents (n=8–9). (c) Liver cholesterol contents (n=8–9). (d) Relative hepatic mRNA levels of genes in HFD-fed mice (n=4–6). (e) Plasma ALT and AST levels (n=10) from HFD-fed Tlr4fl/fland Tlr4LKOmice. *P<0.05, compared between Tlr4fl/fland Tlr4LKOmice on the same diet;#P<0.05, compared between different diets for mice of the same genotype (Student’st-test). All data are presented as means±s.e.m. Figure 4: Hepatocyte Tlr4 promotes the development of hepatic steatosis and liver injury in mice. ( a ) Liver weight in mice fed either chow ( n =8) or HFD ( n =10) for 12 weeks. ( b ) Liver triglyceride contents ( n =8–9). ( c ) Liver cholesterol contents ( n =8–9). ( d ) Relative hepatic mRNA levels of genes in HFD-fed mice ( n =4–6). ( e ) Plasma ALT and AST levels ( n =10) from HFD-fed Tlr4 fl/fl and Tlr4 LKO mice. * P <0.05, compared between Tlr4 fl/fl and Tlr4 LKO mice on the same diet; # P <0.05, compared between different diets for mice of the same genotype (Student’s t -test). All data are presented as means±s.e.m. Full size image Myeloid cell Tlr4 deficiency does not regulate insulin sensitivity To investigate the effect of macrophage Tlr4 in diet-induced obesity and associated metabolic disorders, we generated myeloid-specific Tlr4 null mice (Tlr4 ΔmΦ ) by crossing Tlr4 fl/fl mice to those expressing Cre-recombinase under the control of the myeloid-specific lysozyme M promoter (LysM) [28] . PCR analysis showed that the deleted allele (Tlr4 Δ ) was only observed in peritoneal macrophages, but not in other tissues examined ( Fig. 5a ). Similarly, mRNA expression of Tlr4 was dramatically reduced (>90%) in the peritoneal macrophages of Tlr4 ΔmФ mice ( Fig. 5b ). Analysis of macrophage Tlr4-mediated cytokine production in response to LPS showed that there was an ~ 35% reduction of circulating Tnfα in Tlr4 ΔmФ mice compared with that of chow-fed Tlr4 fl/fl mice ( Fig. 5c,d ). 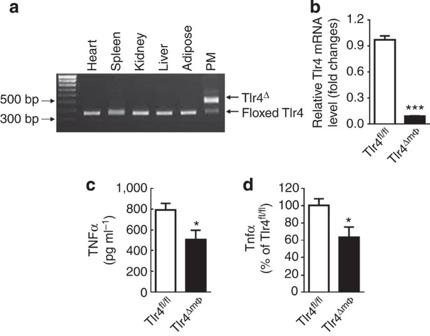Figure 5: Generation of mice lacking Tlr4 in myeloid cells. (a) PCR analysis of genomic DNA isolated from the indicated tissues of 6-week-old Tlr4ΔmΦmice. (b) qPCR analysis of Tlr4 mRNA expression in peritoneal macrophage (PM) isolated from chow-fed mice. (c) LPS (1 mg kg−1body weight) was injected intraperitoneally to chow-fed mice. Blood was collected 1.5 h after LPS administration and plasma Tnfα levels were measured (n=5–6). (d) Levels are presented as a percentage relative to Tlr4fl/fllevels. *P<0.05, ***P<0.001, compared between Tlr4ΔmΦmice and Tlr4fl/flmice (Student’st-test). All data are presented as means±s.e.m. Figure 5: Generation of mice lacking Tlr4 in myeloid cells. ( a ) PCR analysis of genomic DNA isolated from the indicated tissues of 6-week-old Tlr4 ΔmΦ mice. ( b ) qPCR analysis of Tlr4 mRNA expression in peritoneal macrophage (PM) isolated from chow-fed mice. ( c ) LPS (1 mg kg −1 body weight) was injected intraperitoneally to chow-fed mice. Blood was collected 1.5 h after LPS administration and plasma Tnfα levels were measured ( n =5–6). ( d ) Levels are presented as a percentage relative to Tlr4 fl/fl levels. * P <0.05, *** P <0.001, compared between Tlr4 ΔmΦ mice and Tlr4 fl/fl mice (Student’s t -test). All data are presented as means±s.e.m. Full size image Next, we examined whether Tlr4 expression in myeloid cells affected diet-induced adiposity and insulin sensitivity. Regardless of diets, Tlr4 ΔmФ mice had similar body weights as their controls ( Fig. 6a ), and had comparable fat pad weights ( Supplementary Fig. 6a ). In addition, Tlr4 ΔmФ mice developed similar degrees of hyperglycaemia, hyperinsulimia, glucose intolerance and insulin resistance as Tlr4 fl/fl mice ( Fig. 6b–f ). Furthermore, both HFD-fed Tlr4 fl/fl and Tlr4 ΔmФ mice developed fatty liver and had comparable hepatic triglyceride and cholesterol contents ( Supplementary Fig. 6b–d ). These data suggest that macrophage Tlr4 deficiency does not protect mice from diet-induced obesity, insulin resistance or hepatic steatosis. 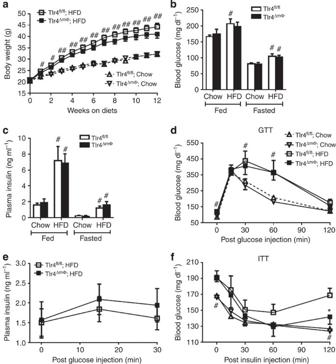Figure 6: Macrophage Tlr4 deficiency does not protect mice from diet-induced obesity or insulin resistance. (a) Body weight curves in Tlr4fl/fland Tlr4ΔmΦmice on a chow (n=9–11) or HFD (n=15) for 12 weeks. (b,c) Blood glucose (b) and plasma insulin (c) concentrations (n=6–8) in Tlr4fl/fland Tlr4ΔmΦmice after 8 weeks of diet feeding under either fed or overnight fasted states. (d) Glucose tolerance test (GTT, 1.5 mg g−1BW,n=5–9 for chow-fed mice;n=8 for mice on HFD) in overnight fasted mice. (e) Glucose-stimulated insulin secretion in overnight fasted HFD-fed mice. Glucose (1.5 mg g−1BW) were injected intraperitoneally and plasma insulin concentrations were measured at the indicated time points (n=8–9). (f) Insulin tolerance test (ITT, 1.5 mU g−1BW,n=5–8 for chow-fed mice;n=11–13 for mice on HFD) in mice fasted for 5 h. *P<0.05, compared between Tlr4fl/fland Tlr4ΔmΦmice on the same diet;#P<0.05,##P<0.01, compared between different diets for mice of the same genotype (Student’st-test). All data are presented as means±s.e.m. Figure 6: Macrophage Tlr4 deficiency does not protect mice from diet-induced obesity or insulin resistance. ( a ) Body weight curves in Tlr4 fl/fl and Tlr4 ΔmΦ mice on a chow ( n =9–11) or HFD ( n =15) for 12 weeks. ( b , c ) Blood glucose ( b ) and plasma insulin ( c ) concentrations ( n =6–8) in Tlr4 fl/fl and Tlr4 ΔmΦ mice after 8 weeks of diet feeding under either fed or overnight fasted states. ( d ) Glucose tolerance test (GTT, 1.5 mg g −1 BW, n =5–9 for chow-fed mice; n =8 for mice on HFD) in overnight fasted mice. ( e ) Glucose-stimulated insulin secretion in overnight fasted HFD-fed mice. Glucose (1.5 mg g −1 BW) were injected intraperitoneally and plasma insulin concentrations were measured at the indicated time points ( n =8–9). ( f ) Insulin tolerance test (ITT, 1.5 mU g −1 BW, n =5–8 for chow-fed mice; n =11–13 for mice on HFD) in mice fasted for 5 h. * P <0.05, compared between Tlr4 fl/fl and Tlr4 ΔmΦ mice on the same diet; # P <0.05, ## P <0.01, compared between different diets for mice of the same genotype (Student’s t -test). All data are presented as means±s.e.m. Full size image Myeloid cell Tlr4 deficiency promotes inflammatory response Next, we examined whether Tlr4 expression in myeloid cells affected diet-induced inflammation. We found that the mRNA expression levels of several pro-inflammatory genes in WAT were not different between the two genotypes on HFD ( Fig. 7a ). Unexpectedly, we found that circulating pro-inflammatory cytokines (Tnfα, IL-6, IL-1β and Mcp1) were dramatically increased in Tlr4 ΔmФ mice on HFD ( Fig. 7b ). Interestingly, we also found that several genes involved in M2 anti-inflammatory markers, such as Arg1, Clec10a and Mrc1, were elevated in WAT of HFD-fed Tlr4 ΔmФ mice ( Fig. 7c ). Consistent with these findings, circulating IL-10 level was also increased in obese Tlr4 ΔmФ mice ( Fig. 7d ). 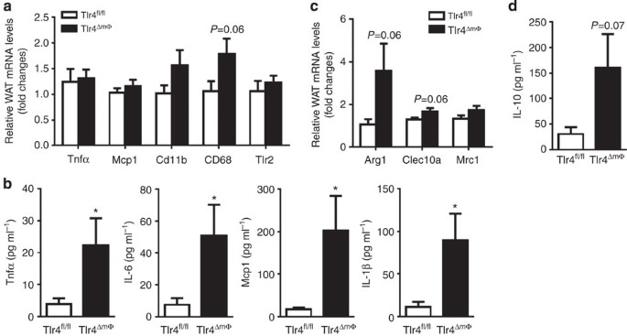Figure 7: Macrophage Tlr4 deficiency results in elevated circulating inflammatory cytokines in obese mice. (a) qPCR analysis of genes in epididymal WAT (n=5–7). (b) Plasma Tnfa, IL-6, IL-1β and Mcp1 levels in mice fed HFD for 12 weeks (n=10–13 for Tnfα, IL-1β and Mcp1;n=6–7 for IL-6). (c) qPCR analysis of genes involved in M2 macrophage activation in epididymal WAT (n=5–7). (d) Plasma IL-10 level in mice on HFD (n=6–7). *P<0.05, compared between Tlr4fl/fland Tlr4ΔmΦmice (Student’st-test). All data are presented as means±s.e.m. Figure 7: Macrophage Tlr4 deficiency results in elevated circulating inflammatory cytokines in obese mice. ( a ) qPCR analysis of genes in epididymal WAT ( n =5–7). ( b ) Plasma Tnfa, IL-6, IL-1β and Mcp1 levels in mice fed HFD for 12 weeks ( n =10–13 for Tnfα, IL-1β and Mcp1; n =6–7 for IL-6). ( c ) qPCR analysis of genes involved in M2 macrophage activation in epididymal WAT ( n =5–7). ( d ) Plasma IL-10 level in mice on HFD ( n =6–7). * P <0.05, compared between Tlr4 fl/fl and Tlr4 ΔmΦ mice (Student’s t -test). All data are presented as means±s.e.m. Full size image Increased SVF Tlr4 expression in mice lacking myeloid cell Tlr4 It has been reported that Tlr4 is highly expressed in adipocytes and obese adipose tissues [9] . Moreover, obese mice show elevated Tlr4 expression in dendritic cells isolated from stromal vascular fraction (SVF) of adipose tissue [29] . In addition, Tlr4 expression is increased in B cells from subjects with inflammatory diseases [30] , [31] . To examine whether Tlr4 expression is upregulated in adipocytes or other cell types in HFD-fed Tlr4 ΔmФ mice, we isolated adipocytes and SVF from obese animals. While Tlr4 mRNA expression in adipocytes was comparable between the two genotypes, its expression in SVF was greatly increased in Tlr4 ΔmФ mice ( Fig. 8a,b ). Expectedly, even after HFD feeding, we observed greatly reduced Tlr4 expression levels in Tlr4 ΔmФ mice compared with that of control mice ( Fig. 8c ). 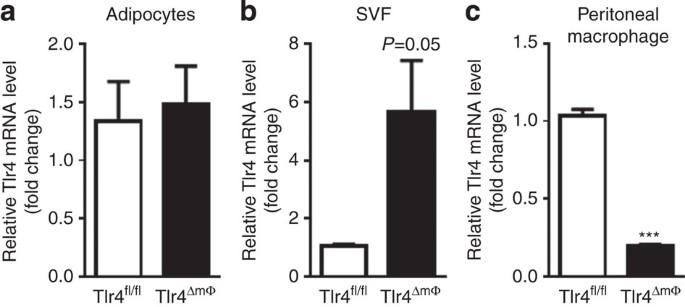Figure 8: Elevated Tlr4 mRNA expression in SVFs of adipose tissues from Tlr4ΔmΦmice. (a,b) qPCR analysis of Tlr4 mRNA expression in the adipocytes (a) and stromal vascular fraction (b, SVF) isolated from epididymal WAT of Tlr4fl/fland Tlr4ΔmΦmice fed HFD (n=3–4). (c) qPCR analysis of Tlr4 mRNA expression in the peritoneal macrophage isolated from Tlr4fl/fland Tlr4ΔmΦmice fed HFD for 12 weeks (n=4). ***P<0.001, compared between Tlr4fl/fland Tlr4ΔmΦmice (Student’st-test). All data are presented as means±s.e.m. Figure 8: Elevated Tlr4 mRNA expression in SVFs of adipose tissues from Tlr4 ΔmΦ mice. ( a , b ) qPCR analysis of Tlr4 mRNA expression in the adipocytes ( a ) and stromal vascular fraction ( b , SVF) isolated from epididymal WAT of Tlr4 fl/fl and Tlr4 ΔmΦ mice fed HFD ( n =3–4). ( c ) qPCR analysis of Tlr4 mRNA expression in the peritoneal macrophage isolated from Tlr4 fl/fl and Tlr4 ΔmΦ mice fed HFD for 12 weeks ( n =4). *** P <0.001, compared between Tlr4 fl/fl and Tlr4 ΔmΦ mice (Student’s t -test). All data are presented as means±s.e.m. Full size image Several lines of evidence have shown that Tlr4 is a critical link mediating obesity-related low-grade inflammation and insulin resistance. However, most of these studies used Tlr4 whole-body knock out or loss-of-function mutant mice. Therefore, the role of Tlr4 in specific tissue(s) in the regulation of inflammation and insulin resistance, both locally and systemically, has remained unclear. In the present study, we found that mice deficient in hepatocyte Tlr4 have an attenuated HFD-induced inflammatory response, in both tissues and in the circulation. Previously, it has been reported that hepatocyte Tlr4 mediates a relatively weak inflammatory response to LPS treatment in vitro [17] . Consistently, after an intraperitoneal injection of LPS in vivo , we observed a ~ 25% reduction of circulating Tnfα in Tlr4 LKO mice compared with that of control mice ( Fig. 1c,d ). Interestingly, despite this relatively low inflammatory response initiated by hepatocytes, we found that HFD-induced chronic, low-grade inflammation was dramatically blunted not only in the liver but also in the adipose tissue and the circulation in Tlr4 LKO mice ( Fig. 3 ). Notably, the HFD-fed Tlr4 LKO mice displayed less hepatic steatosis and enhanced liver function ( Fig. 4 ). Conversely, obese Tlr4 fl/fl mice showed signs of liver injury, and it is likely that inflammatory signalling is amplified through interactions between impaired hepatocytes and activated Kupffer cells. Currently, the mechanism mediating these inter-cell effects is unknown. However, it has been reported that nitric oxide, synthesized by both hepaotcytes and Kupffer cells, may mediate the interactions and regulate hepatic functions [32] . In addition, IL-1α released from chronically damaged hepatocytes could activate neighbouring Kupffer cells, leading to the release of inflammatory cytokines and the subsequent stimulation of compensatory hepatocyte proliferation [33] . Extensive investigations have identified inflammation to be a major contributor in the aetiology of insulin resistance [21] . In the present study, inactivation of hepatocyte Tlr4 results in significantly reduced pro-inflammatory markers in liver, which could partially contribute to the enhanced hepatic insulin sensitivity in obese Tlr4 LKO mice. Some studies have demonstrated that hepatic accumulation of triglyceride and other lipid metabolites, such as ceramide and/or diacylglycerol (DAG), also play critical roles in the development of insulin resistance [34] , [35] . For instance, Holland et al. [36] reported that ceramide is essential for Tlr4-mediated insulin resistance induced by systemic lard oil and fatty acid infusions. In contrast, Galbo et al. [37] showed that the accumulation of DAG, but not Tlr4 signalling or ceramide systhesis, is required for saturated fat-induced hepatic insulin resistance. Thus, reductions in liver triglycerides, ceramides and/or DAG in HFD-fed Tlr4 LKO mice may also contribute to the improved hepatic insulin sensitivity that we observed. Lipid infusions can initiate an acute inflammatory response [36] , and acute administrations of HFD are sufficient to induce hepatic steatosis, but not obesity [37] . It should be noted that in our study, mice were fed HFD for 12 weeks, and developed both steatosis and obesity, which is a key difference from previous studies [36] , [37] . Many studies have focused on the crosstalk between liver and other tissues in the development of obesity-related metabolic disorders. For example, impaired hepatic IL-6 signalling leads to modest insulin resistance in liver, but a more severe defect in insulin action in skeletal muscle and WAT [38] . In addition, it has been shown that a liver-derived secretory protein regulates insulin sensitivity in both liver and muscle [39] . Recently, El Ouaamari et al. [40] reported that hepatocyte-derived factor(s) stimulates β cell proliferation in insulin-resistant states. Collectively, growing lines of evidence indicate that altered hepatocyte metabolism may lead to functional changes in other tissues. In any case, we make the interesting observation that we induce changes along the hepato-adipo axis. While inter-organ crosstalk from the adipocyte to the liver is well established, convincing evidence for powerful hepatokines is more limited. The fact that changes in hepatic Tlr4 prompt profound changes at the level of the macrophage population in adipose tissue could certainly be explained by a hepatokine, even though we cannot exclude that this is a secondary event to systemic improvements in metabolism. Consistent with previous studies showing that Tlr4 global deficient mice have attenuated diet-induced hepatic steatosis [8] , [11] , [23] , [41] , we also found that mice lacking hepatocyte Tlr4 had less hepatic triglyceride contents and reduced mRNA expression of several genes involved in de novo lipogenesis ( Fig. 4 ). Our data indicate that decreased endogenous lipid synthesis could partly contribute to the improved hepatic steatosis. Indeed, it has been shown that low doses of LPS stimulate hepatic endogenous fatty acid synthesis, which are substrates for hepatic triglyceride production [42] . Although we found comparable mRNA expression levels of Acox1, we cannot rule out the contribution of reduced fatty acid oxidation to the reduction in liver triglyceride content seen in obese Tlr4 LKO mice. In addition, it is possible that reduced fat uptake and/or elevated VLDL secretion could contribute to the decreased hepatic fat accumulation in HFD-fed Tlr4 LKO mice. Previous studies have consistently shown that whole-body Tlr4 null mice are protected from diet-induced chronic low-grade inflammation [7] , [8] , [9] , [10] , [11] . Given the important role of macrophages in the generation of inflammatory cytokines and chemokines, and the high expression levels of Tlr4 in macrophages [9] , we expected to observe attenuated inflammatory responses in Tlr4 ΔmФ mice. Surprisingly, we found elevated circulating inflammatory cytokines in Tlr4 ΔmФ mice ( Fig. 7b ). Interestingly, we also found that the SVFs isolated from HFD-fed Tlr4 ΔmФ mice had significantly increased Tlr4 mRNA expression compared with that of control mice ( Fig. 8b ). These results suggest that compensatory increases in Tlr4 expression in other cell types, such as dendritic cells, B cells or endothelial cells, could contribute to the elevated inflammatory response. Consistently, it has been reported that HFD feeding promotes the upregulation of Tlr4 expression in SVF of adipose tissue [29] . Furthermore, Tlr4 expression is modestly increased in B cells isolated from subjects with inflammatory diseases [30] , [31] . In vitro experiments show that macrophage Tlr4 mediates a potent immune response. However, we only observed a ~ 35% reduction of circulating Tnfα levels in Tlr4 ΔmФ mice after intraperitoneal LPS treatment ( Fig. 5c,d ), indicating that other Tlr4-expressing cells likely contribute to the LPS-induced inflammatory response. Despite the increased inflammatory response seen in obese Tlr4 ΔmФ mice, we observed comparable impaired glucose homeostasis and insulin resistance between HFD-fed Tlr4 ΔmФ and Tlr4 fl/fl mice ( Fig. 6 ). This could be due to the increased M2 anti-inflammatory markers in the WAT and in the circulation (IL-10) ( Fig. 7 ), which would compensate for the pro-inflammatory cytokine-mediated insulin resistance. Indeed, accumulating evidence has shown that alternative macrophage activation plays an important role in improving insulin sensitivity [21] , [43] , [44] . Of note, it has been reported that both global and hematopoietic cell Tlr4 deficiency promote the alternative activation of adipose tissue macrophages [23] . Despite our observation that myeloid cell-specific deletions of Tlr4 did not modulate whole-body insulin sensitivity, we cannot rule out the critical role of macrophage-induced inflammation (pro- or anti-) in the development of insulin resistance. What is important to note is that we present here for the first time a model of Cre-LoxP technology-mediated elimination of the Tlr4 gene. The observations reported are made in a fundamentally different setting from the whole-body knock out or from bone marrow transplant-based models. Our macrophage-based knock out animals leave the potential open for a compensatory upregulation of Tlr4 in other stromal vascular cells, whereas the bone marrow transplant-based approach may be more limited in its ability to do that. Similarly, the hepatocyte-specific null may offer an opportunity for altered Tlr4 levels in other hepatic cell types, whereas the whole-body knock out lacks that option for compensation. Collectively, our data suggest that Tlr4s expressed by hepatocytes play a physiologically important role in regulating obesity-induced metabolic disorders including inflammation, insulin resistance and hepatic steatosis. These findings may also help elucidate novel strategies for the treatment of the metabolic syndrome by specifically targeting hepatocyte Tlr4s. Mice To generate mice bearing a Cre-conditional Tlr4 null allele, a BAC clone (bMQ58F22 from Sanger Institute) containing the murine Tlr4 gene derived from the 129/Sv strain was electroporated into EL350 bacteria. First, the loxP sequence present in the BAC backbone was removed and replaced with a Zeocin gene by homologous recombination using pZErO-1 Vector (Invitrogen) [45] . Next, the loxP-Kanamycin-loxP cassette was amplified from pL452 using primers 5′-TAAGATGTCTTGCAAATATGAAGAGGCAGATAAATAAATGGAGAAGGATGGGTGTGATACGCCTCCCTGGCTTCCGATCATATTCAATAACCC-3′ and 5′-TTAGCTATACAGTCAAAGATAACATTGGACTCCCAAAATACCTGCCATTCTGGGGATATGGTGGATCCCCTCGAGGGACC-3′ and the amplicon was used for homologous recombination. Kanamycin-resistant clones were selected and recombination was verified by PCR. Following this, expression of Cre-recombinase was induced, which allowed for the recombination of the loxP sites and removal of the Kanamycin gene. Then, the Frt-Kanamycin/Neomycin-Frt-loxP cassette was amplified from pL451 using primers 5′-AGCAGATGCATAAAGGTGGAGGTTTTTTATTGTAAGTGAAATATGCCAGGCACAGAAGGAACTCACTATAGGGCGAATTGG-3′ and 5′-GTTCTGCATATTATTTTTTCTAACTTTGCTCATGTCATCAAAAGTTCCTGAAAGGCCAGTAGCACTGCTCTAGAACTATGTGATCCTC-3′ and the amplicon was used for homologous recombination. Clones resistant to kanamycin were selected and recombination was verified by PCR. EL350 clones containing the correctly modified BAC Tlr4 sequence were confirmed by PCR analysis and DNA sequencing. BAC DNA was isolated using the Plasmid Midi Kit (Qiagen) and linearized with NotI for electroporation into 129/SvJ ES cells by the transgenic core facility at the University of Texas Southwestern Medical Center. Neomycin-resistant clones were selected and genomic DNA was isolated for a custom multiplex TaqMan quantitative PCR (qPCR) assay to identify the recombinant clones. Briefly, extracted DNA was used as template (5–100 ng). Melanocortin 4 receptor (MC4R) was used as an endogenous reference (ID Mm00457483_s1, FAM dye-labelled probe; Applied Biosystems). Primers and probe (Biosearch Technologies, Novato) used to screen the loxP-flanked Tlr4 allele were as follows: forward primer: 5′-TCTTGCAAATATGAAGAGGCAGATA-3′; reverse primer: 5′-GACCAGTCTGGCCTTAAATTAGC-3′; and VIC dye-labelled probe: 5′-TGTGATACCATATCCCCAGAATG-3′. DNA-based qPCR reactions were conducted on an Applied Biosystems PRISM 7900HT sequence detection system. To distinguish the targeted ES cell clones, we calculated the ΔCT as the difference between the CT values of the custom and the reference qPCRs, and the average WT ΔCT. Individual ΔΔCT values were calculated by subtracting the average WT ΔCT from the individual ΔCT. ES cell clones with ΔΔCT values more than 0.5 were considered to be targeted. The recombinant ES cells were injected into blastocysts of C57 mice. Chimeric male mice (F0) were crossed to C57BL/6 female mice and brown pups (F1) were screened for germ line transmission by PCR (using the same strategy as for genotyping). F1 pups carrying the Cre-conditional Tlr4 null allele Tlr4 fl/wt were then mated to FLPe recombinase (Flp) transgenic mice to induce the recombination of the Frt sites and removal of Kanamycin/Neomycin gene. Tlr4 fl/wt mice ubiquitously expressing Flp transgene (F2) were confirmed by PCR. These F2 mice were then crossed with one of the three transgenic mice: (1) Zona Pellucida 3 (Zp3)-Cre transgenic mice to generate mice lacking Tlr4 in all tissues (Tlr4 KO ), (2) Albumin-Cre transgenic mice to produce mice lacking Tlr4 in hepatocytes (Tlr4 LKO ) and (3) LysM-Cre mice to generate mice lacking Tlr4 in myeloid cells (Tlr4 ΔmΦ ). Mice bearing a WT and/or floxed Tlr4 allele (Tlr4 fl/fl ) were genotyped by primer pairs P1 (5′-GACTTGAGAGTTATGTAACACCTGA-3′) and P2 (5′-TCCTATAGACCAGTCTGGCCTTAA-3′). Primers P1 and P3 (5′-GTGGCTATGTTCCAGTTTGAATG-3′) were used to screen the Tlr4 Δ allele. Animal care and diets Animals were housed in a temperature-controlled environment on a 12-hour light/12-hour dark cycle. They were fed either standard chow (2916 Global Diet; Harlan Teklad) or HFD (TD. 88137 Western Diet; Harlan Teklad). Mice were backcrossed into C57BL/6 background for at least three generations. Only male mice were used in the present experiments. Care of all animals and procedures were approved by the Institutional Animal Care and Use Committee of the University of Texas (UT) Southwestern Medical Center at Dallas. Endotoxin-induced inflammatory response Chow-fed WT and Tlr4 KO mice (6–8 weeks old) were treated with LPS (1 mg kg −1 body weight (BW), O55:B5; Sigma) by intraperitoneal injection. Similarly, chow-fed, 7–10 week-old Tlr4 ΔmΦ , Tlr4 LKO and their littermate control mice were administered 1 mg kg −1 BW of LPS. Blood was collected 1.5 h after injection by tail bleeding. Plasma Tnfα concentrations were determined using the MILLIPLEX MAP Mouse Cytokine/Chemokine-Premixed 32 Plex assay (Millipore). Glucose and insulin tolerance tests GTTs were performed in mice that were fed either chow or HFD for 9 weeks. One week later, the same mice were used for ITT. For GTT, mice were fasted for 5 h or overnight (16 h). After measuring the baseline blood glucose level via a tail nick using a glucometer (Alpha TRAK), 1.2 mg g −1 BW or 1.5 mg g −1 BW of glucose was injected intraperitoneally. Blood glucose levels were then measured at 15, 30, 60 and 120 min after glucose injection. For ITT, 5-h fasted mice were injected intraperitoneally with recombinant human insulin (Eli Lilly) at 1.5 mU g g −1 BW and their blood glucose concentrations (before and at 15, 30, 60 and 120 min post insulin administration) were determined from tail blood using a glucometer. Glucose-stimulated insulin secretion After 10 weeks of HFD feeding, Tlr4 fl/fl and Tlr4 LKO mice were fasted overnight and glucose was injected into the peritoneal cavity at 2 mg g −1 BW. Blood samples were collected at 0, 15 and 30 min from mouse tails and plasma insulin concentrations were measured using an ELISA kit (Crystal Chem, Inc.). Tissue histology Adipose tissues were fixed in buffered 10% formalin and processed for hematoxylin and eosin (H&E) staining by the Molecular Pathology Core at UT Southwestern Medical Center. For immunohistochemistry (IHC), sections were deparaffinized. After antigen retrieval and blockage of endogenous peroxidase, sections were stained with primary antibodies against Mac2 (1:1,000, CEDARLANE Labs) followed by biotinylated secondary anti-rabbit antibody (1: 500, Dako). Secondary antibodies were detected using a DAB chromogen A kit (Dako) according to the manufacturer’s instructions. The slides were also counterstained with haematoxylin. All the images were visualized and captured with a Zeiss microscope (Imager ZI) equipped with a digital camera (Axiocam). Liver lipid contents After a 4-h fast, mice were killed and livers were removed and snap-frozen in liquid nitrogen and stored at −80 °C. Frozen liver tissues were used for lipid extraction by the UT Southwestern Mouse Metabolic Phenotyping Core Facility. After extraction, triglyceride and cholesterol contents were measured using Infinity Reagent assays (Thermo Fisher Scientific). Plasma parameters Animals were killed and blood was collected in EDTA-coated tubes. After centrifugation at 6,000 g for 15 min, plasma was separated and stored at −80 °C. Plasma triglyceride, cholesterol, free fatty acids, AST and ALT concentrations were measured using the Vitros 250 Chemistry Analyzer (Ortho Clinical Diagnostics). Plasma leptin and insulin were determined by Mouse Leptin ELISA and Ultra-Sensitive Mouse Insulin ELISA Kits (Crystal Chem, Inc.), respectively. Blood glucose concentrations from tail blood were measured with a glucometer and glucose strips (Alpha TRAK). Hyperinsulinemic–euglycemic clamp study After 16 weeks of HFD feeding, Tlr4 fl/fl and Tlr4 LKO mice were cannulated via the jugular vein and allowed to recover for 1 week. On the day of the experiment, 4-h-fasted mice were infused with [3- 3 H]-glucose (5 μCi bolus followed by 0.05 μCi min −1 ) to measure glucose turnover at t =−120 min. At t =−15 and −5 min, blood samples from the cut tail were taken for measurements of basal insulin and glucose as well as to calculate glucose turnover. The clamp was started at t =0 min with a continuous insulin infusion (10 mU kg −1 min −1 ; Humulin, Eli Lilly), and the [3- 3 H]-glucose was increased to 0.1 μCi min −1 to minimize changes in specific activity. A variable glucose infusion rate (50% dextrose) was used to maintain blood glucose at 150 mg dl −1 . Blood samples were taken every 10 min during the steady-state period ( t =80–120 min) to determine hepatic glucose production and glucose disposal rate. Western blot of insulin signalling in WAT After 12 weeks of HFD feeding, Tlr4 fl/fl and Tlr4 LKO mice were fasted overnight. Saline or 5U kg −1 BW of recombinant human insulin (Eli Lilly) were injected intraperitoneally. Ten minutes later, epidydimal fat pads were quickly removed and snap-frozen in liquid nitrogen. Tissues were stored at −80 °C. For analysis of insulin-stimulated Akt/protein kinase B (PKB) phosphorylation, tissues were homogenized in RIPA lysis buffer (Sigma) containing protease inhibitors (P2714, Sigma) and phosphatase inhibitor (PI-78420,Thermo Scientific), followed by solubilization and centrifugation at 12,000 r.p.m. for 15 min at 4 °C. Supernatants were stored at −80 °C until assays were performed. Tissue protein concentrations were determined by bicinchoninic acid (BCA) Kit (Pierce) and fractionated on a SDS-PAGE gel. Proteins were transferred to a nitrocellulose membrane by electroblotting, and membranes were blocked in TBS containing 0.05% Tween 20 and 5% nonfat milk, and incubated with rabbit anti-phospho-Akt/PKB antibody (Ser473, Cell Signaling Technology) at 1: 2,000 dilution in 5% BSA overnight, followed by anti-rabbit IgG (1:10,000, Jackson Immunoresearch Lab.) in blocking solution for 1 h. After incubation with ECL (Pierce), the membranes were exposed to X-ray films for image development. After stripping the membrane, the same membrane was used for the detection of total Akt/PKB (1: 2,000, Cell Signaling Technology). qPCR Mice were killed after 12 weeks of HFD feeding, and tissues were quickly removed, snap-frozen in liquid nitrogen and stored at −80 °C. Total RNAs from liver and WAT were extracted using RNA Stat60 (Teltest). Complementary DNA was synthesized using the High Capacity cDNA Kit (Applied Biosystems). Primers for Tlr4 (ID: Mm0445273_m1), Socs3 (ID: Mm00545913_s1), Cd11c (ID: Mm00498698_m1), Foxo1 (ID: Mm00490672_m1), Pepck (ID: Mm00440636_m1), Acox1 (ID: Mm01246831_m1), CD68 (ID: Mm03047340_m1) and Tlr2 (ID: Mm00442346_m1) were purchased from Applied Biosystems. Primers sequences for other genes shown in the paper are listed as follows: Tnfα, forward, CTGAGGTCAATCTGCCCAAGTAC, and reverse, CTTCACAGAGCAATGACTCCAAAG; Mcp1, forward, TTTTTGTCACCAAGCTCAAGAGA, and reverse, ATTTGGTTCCGATCCAGGTT; IL-6, forward, TCGTGGAAATGAGAAAAGAGTTG, and reverse, AGTGCATCATCGTTGTTCATACA; IL-1β, forward, TGACGGACCCCAAAAGATG, and reverse, TGGACAGCCCAGGTCAAAG; Cd11b, forward, ATCAACACAACCAGAGTGGATTC, and reverse, GTTCCTCAAGATGACTGCAGAAG; Acc1, forward, TGGACAGACTGATCGCAGAGAAAG, and reverse, TGGAGAGCCCCACACACA; Fas, forward, GCTGCGGAAACTTCAGGAAAT, and reverse, AGAGACGTGTCACTCCTGGACTT; Scd1, forward, CCGGAGACCCCTTAGATCGA, and reverse, TAGCCTGTAAAAGATTTCTGCAAACC; Arg1, forward, AGACCACAGTCTGGCAGTTG, and reverse, CCACCCAAATGACACATAGG; Mrc1, forward, TGATTACGAGCAGTGGAAGC, and reverse, GTTCACCGTAAGCCCAATTT; Clec10a, forward, CTCTGGAGAGCACAGTGGAG, and reverse, ACTTCCGAGCCGTTGTTCT. mRNA contents were normalized to 18s mRNA levels. All assays were performed using an ABI Prism 7900HT sequence detection system (Applied Biosystems). The relative amounts of all mRNAs were calculated using the ΔΔCT assay. Primary hepatocyte and peritoneal macrophage isolation For primary hepatocyte isolation, mice were anaesthetized, and livers were perfused with 30 ml of Liver Perfusion Medium (Gibco) and then with 30 ml of Liver Digestion Medium (Gibco) at a rate of 3 ml min −1 via the portal vein. After the perfusion and digestion at 37 °C, the livers were removed, the hepatic capsule was peeled off, and hepatocytes were dispersed by shaking the digested liver in Liver Digestion Medium at 37 °C, followed by filtration through gauze. Digestion was stopped by the addition of an equal volume of ice-cold Dulbecco's modified Eagle medium (DMEM) containing 5% ( v / v ) fetal bovine serum (FBS), 10 mM Hepes (pH 7.4), 100 U ml −1 penicillin and 100 μg ml −1 streptomycin. The cells were washed twice and resuspended in the same medium. Cell viability, determined by trypan blue dye exclusion, was 90–95%. The cells were plated on 60- or 35-mm dishes coated with mouse type IV collagen in the above medium at a density of 1.5 × 10 6 cells or 0.5 × 10 6 cells per dish, respectively. After incubation for 2 h (period of attachment), the cells were washed and then used for experiments. To isolate peritoneal macrophage, 3-month-old chow-fed mice were injected with 2 ml of 3% thioglycolate. Four days later, mice were anaesthetized and elicited peritoneal macrophages were isolated from the peritoneal cavity. After centrifugation at 1,000 r.p.m. for 10 min at 4 °C, cell pellets were resuspended and seeded in six-well plates in RPMI 1640 medium containing 10% FBS, 100 U ml −1 penicillin and 100 μg ml −1 streptomycin. Two hours later, cells were washed by phosphate-buffered saline (PBS), and adherent macrophages were used for genomic DNA or RNA isolation. Adipocyte and SVF isolation Epididymal fat pads were collected from Tlr4 fl/fl and Tlr4 ΔmΦ mice fed HFD for 11 weeks. Tissues were minced and digested using collagenase (Gibco, #17703-034) at 37 °C for 1.5 h with shaking. The cell suspension was filtered through a 250-μm mesh, washed with DMEM containing 10% FBS, and centrifuged at 800 g for 1 min at room temperature. The floating adipocytes were collected, centrifuged at 500 g for 1 min and dissolved in TRIzol for RNA isolation. The remaining cell pellets containing SVF were put on ice immediately. The pellets were passed through 40-μm cell strainer, washed with cold DMEM buffer and centrifuged at 500 g for 5 min at 4 °C. Then, SVF were collected as pellets and resuspended in TRIzol for RNA isolation. Statistical analyses All the results are presented as means±s.e.m. Differences between two groups were determined for statistical significance by a standard two-tailed Student’s t -test. Significance was accepted at a value of P <0.05. How to cite this article: Jia, L. et al. Hepatocyte Toll-like receptor 4 regulates obesity-induced inflammation and insulin resistance. Nat. Commun. 5:3878 doi: 10.1038/ncomms4878 (2014).